EphrinB2 affects apical constriction inXenopusembryos and is regulated by ADAM10 and flotillin-1 The Eph/ephrin signalling pathways have a critical function in cell adhesion and repulsion, and thus play key roles in various morphogenetic events during development. Here we show that a decrease in ephrinB2 protein causes neural tube closure defects during Xenopus laevis embryogenesis. Such a decrease in ephrinB2 protein levels is observed on the loss of flotillin-1 scaffold protein, a newly identified ephrinB2-binding partner. This dramatic decline in ephrinB2 protein levels on the absence of flotillin-1 expression is specific, and is partly the result of an increased susceptibility to cleavage by the metalloprotease ADAM10. These findings indicate that flotillin-1 regulates ephrinB2 protein levels through ADAM10, and is required for appropriate neural tube morphogenesis in the Xenopus embryo. The ephrins are all membrane-bound proteins subdivided into two classes, the A subclass being glycosylphosphatidylinositol-linked to the membrane and the B subclass being transmembrane proteins with a short cytoplasmic domain. The cognate Eph receptors are transmembrane receptor tyrosine kinases, and are also divided into two classes (A and B) based on their sequence similarity and their binding specificity towards the ephrin subclasses. Eph-ephrin contact dependent interactions between two cells result in bi-directional signalling. During development, these Eph/ephrin interactions lead to cell sorting and boundary formation between receptor and ligand-bearing cells [1] . When motile cells expressing either Eph or ephrin come in contact with cells expressing the cognate partner, the response is often adhesion or repulsion. The choice between cell adhesion/attraction or de-adhesion/repulsion depends on the cell type and signalling context [2] . In the latter case, Eph/ephrin-mediated adhesion can be released by endocytosis of the Eph/ephrin complex into either Eph- or ephrin-expressing cells, allowing the cells to move on to their respective destination. This endocytosis can be accomplished by ephrinB or EphB transendocytosis [3] , [4] , [5] . The EphB/ephrinB complex is endocytosed in an EphB kinase-dependent manner, preferentially into cells with more adhesive contacts with the substrate and a well-developed actin cytoskeleton [3] . Loss of cell adhesion initiated by EphB/ephrinB is observed during developmental processes such as notochord formation where in response to non-canonical Wnt signalling, phosphorylated EphB receptors make a ternary complex with the scaffold protein dishevelled2 and the formin homology protein Daam1, which is transported to the endocytic vesicles in a dynamin-dependent manner. This removal of EphB molecules from the cell surface results in loss of adhesion, leading to initiation of convergent extension cell movements during notochord development [6] . One critical factor when considering Eph/ephrin-mediated cell repulsion and disengagement is that the interaction between Eph receptors and ephrin proteins must first be terminated. While endocytosis certainly offers a long-term solution to this termination [7] , another efficient way to cease the adhesion is by ectodomain cleavage. A disintegrin and metalloprotease (ADAM) proteins are type I transmembrane proteins with an extracellular metalloproteinase domain and disintegrin and cysteine-rich domains [8] , [9] . ADAMs have been shown to cleave ephrinA and ephrinB proteins [7] , [10] , [11] , and Eph receptors are also subject to cleavage by metalloproteases and γ-secretase [12] , [13] . However, little is known about the mechanisms that control the cleavage of the ephrins and Ephs by these metalloproteases. Here we show that loss of the ephrinB2 interactor, flotillin-1, leads to a marked increase in ephrinB2 protein cleavage and processing, which causes neural tube closure defects in Xenopus embryos and an associated disruption of cell shape and actin cytoskeleton. Moreover, we identify ADAM10 as the specific metalloprotease that cleaves ephrinB2 in the absence of flotillin-1. Thus, we show that ephrinB2 protein levels are sustained by a lipid raft protein (flotillin-1) that interacts with ephrinB2, and inhibits cleavage and processing by ADAM10. Moreover, this study provides a link between ephrinB2 regulation and the important developmental process of neural tube closure. EphrinB2 associates with flotillin-1 EphrinBs have several interacting proteins that mediate or regulate their morphogenetic functions during development [14] . Identifying these regulators in the context of various morphogenetic events and systems can reveal regulatory networks that may function in other cellular contexts. We recently identified the lipid raft protein flotillin-2 as an ephrinB1 interactor by mass spectrometric analysis of immune complexes from Xenopus embryos overexpressing ephrinB1. On the basis of these results, we tested whether ephrinB2 was able to interact with flotillin-1 and flotillin-2 since the intracellular domains of ephrinB1 and ephrinB2 are 82% identical and flotillin-1 and flotillin-2, similar to the ephrinBs, are known to be expressed in the neural tissue in vivo [15] , [16] , [17] . Flag-tagged ephrinB2 and haemagglutinin (HA)-tagged flotillin-1a or -1b were overexpressed in Xenopus oocytes, and co-immunoprecipitation (co-IP) analysis was performed. Flotillin-1a-HA and flotillin-1b-HA were detected in ephrinB2-Flag immune complexes, and ephrinB2-Flag was detected in flotillin-1a- and -1b-HA immune complexes ( Fig. 1a ). Similarly, co-IP analysis of oocytes overexpressing flotillin-2 with ephrinB1 or ephrinB2 also showed an association of both ephrinBs with flotillin-2 ( Supplementary Fig. 1a ). In HT-29 colon carcinoma cells, we were able to co-immunoprecipitate endogenous flotillin-1 with ephrinB2 immune complexes ( Fig. 1b ), confirming that ephrinB2 and flotillin-1 associate in vivo . In addition, we show by in situ hybridization that expression of ephrinB2 , flotillin-1a and flotillin - 1b overlap in the neural plate of neurula stage embryos ( Supplementary Fig. 1b ), as has been shown by others [17] , [18] . Whole mount immunocytochemistry analysis confirmed the expression of flotillin-1 in the neuroepithelium and ectoderm ( Fig. 1c ), where ephrinB2 is known to be expressed ( Supplementary Fig. 1b ; (refs 18 , 19 ), and also shows expression in the somites, notochord and the roof of the archenteron ( Fig. 1c ). 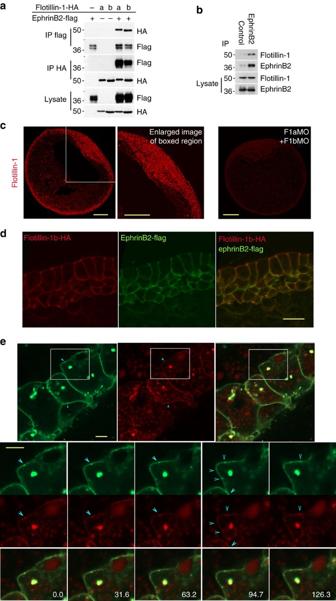Figure 1: EphrinB2 is associated and co-localized with flotillin-1. (a) Flotillin-1 is associated with ephrinB2. Co-IP and western blot analysis ofXenopusoocytes exogenously expressing ephrinB2-Flag with flotillin-1a-HA or -1b-HA. (b) Endogenous ephrinB2 interacts with endogenous flotillin-1. Endogenous ephrinB2 was immunoprecipitated with anti-goat ephrinB2 antibody in HT-29 colon carcinoma cells, and flotillin-1 was detected using anti-mouse flotillin-1 antibody in ephrinB2 immune complexes by western blotting. (c) Flotillin-1 immunostaining of embryo sections. Immunostaining of endogenous flotillin-1 in stage 15 embryos, and a magnified view of the neural plate region. Embryos were also injected with F1aMO and F1bMO as indicated, and immunostained for flotillin-1. Scale bar, 200 μm. (d) Subcellular localization of flotillin-1b-HA and ephrinB2-Flag. Flotillin-1b-HA and ephrinB2-Flag RNA was injected intoXenopusembryos and stained with anti-HA or anti-Flag antibodies. Scale bar, 20 μm. (e) Co-localization of ephrinB2-mCherry and flotillin-1-GFP at the plasma membrane in embryos. Flotillin-1-GFP (green) and ephrinB2-mCherry (red) RNAs were injected into embryos and localization of proteins was observed by confocal microscopy. The merged image is visible as yellow staining. The enlarged images are split screen enlargements of the boxed areas (from different frames of theSupplementary Movie 1) with flotillin-1-GFP (green) at top of split and ephrinB2-mCherry (red) at bottom. Blue arrows indicate the same areas of co-localization in the membrane during movement. Scale bar, 10 μm. Figure 1: EphrinB2 is associated and co-localized with flotillin-1. ( a ) Flotillin-1 is associated with ephrinB2. Co-IP and western blot analysis of Xenopus oocytes exogenously expressing ephrinB2-Flag with flotillin-1a-HA or -1b-HA. ( b ) Endogenous ephrinB2 interacts with endogenous flotillin-1. Endogenous ephrinB2 was immunoprecipitated with anti-goat ephrinB2 antibody in HT-29 colon carcinoma cells, and flotillin-1 was detected using anti-mouse flotillin-1 antibody in ephrinB2 immune complexes by western blotting. ( c ) Flotillin-1 immunostaining of embryo sections. Immunostaining of endogenous flotillin-1 in stage 15 embryos, and a magnified view of the neural plate region. Embryos were also injected with F1aMO and F1bMO as indicated, and immunostained for flotillin-1. Scale bar, 200 μm. ( d ) Subcellular localization of flotillin-1b-HA and ephrinB2-Flag. Flotillin-1b-HA and ephrinB2-Flag RNA was injected into Xenopus embryos and stained with anti-HA or anti-Flag antibodies. Scale bar, 20 μm. ( e ) Co-localization of ephrinB2-mCherry and flotillin-1-GFP at the plasma membrane in embryos. Flotillin-1-GFP (green) and ephrinB2-mCherry (red) RNAs were injected into embryos and localization of proteins was observed by confocal microscopy. The merged image is visible as yellow staining. The enlarged images are split screen enlargements of the boxed areas (from different frames of the Supplementary Movie 1 ) with flotillin-1-GFP (green) at top of split and ephrinB2-mCherry (red) at bottom. Blue arrows indicate the same areas of co-localization in the membrane during movement. Scale bar, 10 μm. Full size image Immunocytochemistry was also performed on embryos injected with antisense morpholino oligonucleotides (MOs) embryos against flotillin-1a and flotillin-1b (F1aMO and F1bMO). The F1aMO- and F1bMO-injected embryos show a dramatic decrease in flotillin-1 immunoreactivity, confirming the specificity of the immunostaining as well as the ability of these MOs to inhibit translation of the endogenous flotillin-1 paralogues ( Fig. 1c ). Moreover, exogenously expressed flotillin-1b-HA and ephrinB2-Flag are both detected in the cell membrane ( Fig. 1d ), suggesting that they are spatially co-localized. In addition, using live cell imaging in embryos co-expressing an ephrinB2-mCherry fusion construct along with a flotillin-1-enhanced green fluorescent protein (EGFP) fusion protein shows that ephrinB2 and flotillin-1 can be found co-localizing on the cell surface ( Fig. 1e ; Supplementary Movie 1 ). Altogether, these data suggest that ephrinB2 and flotillin-1 interact in vivo and may function together during Xenopus development. Loss of flotillin-1 leads to a reduction in ephrinB2 levels Since ephrinB2 is normally localized to the basolateral region of plasma membranes, we examined whether flotillin-1 influences ephrinB2 localization or expression ( Fig. 2a–c ). EphrinB2 RNA was injected into both sides of an embryo, and the F1aMO or F1bMO along with GFP RNA was introduced into only one side. Surprisingly, ephrinB2 protein levels were greatly reduced in the plasma membrane of F1aMO- and F1bMO-bearing cells, as evidenced by the dramatically reduced ephrinB2 fluorescence (red) found in the F1MO-bearing cells (green) when compared with control MO (CoMO)-bearing cells (non-green; Fig. 2b,c ). Western blot analysis also showed that ephrinB2-HA protein expression was greatly diminished when flotillin-1a was knocked down, while exogenous expression of ephrinB1 and ephrinB3 was comparable in the presence of F1aMO or CoMO ( Fig. 2d ). Moreover, the introduction of MO-resistant flotillin-1a or -1b RNA along with the respective MO rescued ephrinB2 protein levels ( Fig. 2e,f ), indicating that flotillin-1 specifically inhibits the loss of ephrinB2 protein expression. 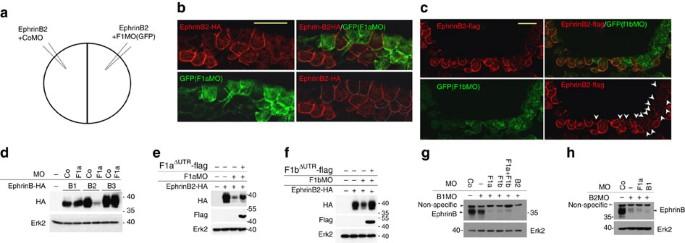Figure 2: Loss of flotillin-1 leads to a reduction in ephrinB2 expression. (a) Injection scheme. CoMO with ephrinB2 RNA is injected into one cell of two-cell-stage embryos, and F1MO along with ephrinB2 RNA and GFP RNA were injected into the other cell. (b) EphrinB2 expression is reduced in the absence of flotillin-1a. F1aMO, ephrinB2-HA RNA and GFP RNA co-injected cells are green. CoMO and ephrinB2-HA RNA-co-injected cells are not green. EphrinB2-HA expression is visualized in red. Cells containing F1aMO, but displaying reduced ephrinB-HA expression are outlined in white dots. Scale bar, 20 μm. (c) F1bMO decreases ephrinB2 expression. F1bMO, ephrinB2-Flag RNA and GFP RNA co-injected cells fluoresce green. CoMO and ephrinB2-Flag RNA-co-injected cells are not green. EphrinB2-HA expression is visualized in red. Arrowheads indicate GFP-expressing cells that harbour the F1bMO. Scale bar, 20 μm. (d) Flotillin-1 knockdown specifically causes ephrinB2 loss. Embryos were injected with HA-tagged ephrinB1, -B2 or -B3 RNAs along with either CoMO or F1aMO. Western blot analysis was performed with anti-HA antibody and anti-Erk2 as a loading control. (e) EphrinB2 loss due to the F1aMO is rescued by re-expression of flotillin-1a. Western blot analysis of embryos injected with ephrinB2-HA RNA and F1aMO, with or without F1aΔUTR-Flag RNA. (f) Decrease in ephrinB2 due to F1bMO is rescued by F1bΔUTR-Flag expression. Western blot analysis of embryos injected with ephrinB2-HA RNA and F1bMO, with or without F1bΔUTR-Flag RNA. (g) Western blot analysis of endogenous ephrinB2 protein in neural folds that have been injected with the indicated MOs, and blotted using the indicated antibodies. Erk2 is used as a loading control. (h) Western blot analysis of endogenous ephrinB1 protein in neural folds that have been injected with the indicated MOs, and blotted using the indicated antibodies. Erk2 is used as a loading control. Figure 2: Loss of flotillin-1 leads to a reduction in ephrinB2 expression. ( a ) Injection scheme. CoMO with ephrinB2 RNA is injected into one cell of two-cell-stage embryos, and F1MO along with ephrinB2 RNA and GFP RNA were injected into the other cell. ( b ) EphrinB2 expression is reduced in the absence of flotillin-1a. F1aMO, ephrinB2-HA RNA and GFP RNA co-injected cells are green. CoMO and ephrinB2-HA RNA-co-injected cells are not green. EphrinB2-HA expression is visualized in red. Cells containing F1aMO, but displaying reduced ephrinB-HA expression are outlined in white dots. Scale bar, 20 μm. ( c ) F1bMO decreases ephrinB2 expression. F1bMO, ephrinB2-Flag RNA and GFP RNA co-injected cells fluoresce green. CoMO and ephrinB2-Flag RNA-co-injected cells are not green. EphrinB2-HA expression is visualized in red. Arrowheads indicate GFP-expressing cells that harbour the F1bMO. Scale bar, 20 μm. ( d ) Flotillin-1 knockdown specifically causes ephrinB2 loss. Embryos were injected with HA-tagged ephrinB1, -B2 or -B3 RNAs along with either CoMO or F1aMO. Western blot analysis was performed with anti-HA antibody and anti-Erk2 as a loading control. ( e ) EphrinB2 loss due to the F1aMO is rescued by re-expression of flotillin-1a. Western blot analysis of embryos injected with ephrinB2-HA RNA and F1aMO, with or without F1a ΔUTR -Flag RNA. ( f ) Decrease in ephrinB2 due to F1bMO is rescued by F1b ΔUTR -Flag expression. Western blot analysis of embryos injected with ephrinB2-HA RNA and F1bMO, with or without F1b ΔUTR -Flag RNA. ( g ) Western blot analysis of endogenous ephrinB2 protein in neural folds that have been injected with the indicated MOs, and blotted using the indicated antibodies. Erk2 is used as a loading control. ( h ) Western blot analysis of endogenous ephrinB1 protein in neural folds that have been injected with the indicated MOs, and blotted using the indicated antibodies. Erk2 is used as a loading control. Full size image We examined the endogenous ephrinB1 and ephrinB2 protein expression in the presumptive neural tube of F1aMO-injected embryos, since this region shows robust overlap in expression of the ephrinB and flotillin-1 genes ( Supplementary Fig. 1b ). Since the ephrinB antibody has cross-reactivity to all three ephrinBs, the F1aMO-injected embryos were co-injected with either ephrinB1MO (B1MO) and/or ephrinB2 MO (B2MO) to detect the remaining ephrinB isoform. The dorsal axial region (neural fold) of these embryos was excised and subjected to western analysis ( Fig. 2g ). The analysis shows that injection of both B1MO and B2MO blocks almost all detectable ephrinB signal in the dorsal axial region, indicating that most of the detectable ephrinB protein is due to ephrinB1 and ephrinB2 ( Fig. 2g ). As expected, when B1MO-harbouring embryos are co-injected with F1aMO or F1bMO, a dramatic loss of the endogenous ephrinB2 protein is observed in the dorsal axial region ( Fig. 2g ). In contrast, co-injection of F1aMO in B2MO-bearing embryos shows only a very modest effect on the relatively low level of ephrinB1 protein found in this tissue ( Fig. 2h ). These data indicate that endogenous ephrinB2 protein is preferentially decreased in neural tissue in the absence of flotillin-1. EphrinB2 ectodomain is critical for decreased ephrinB2 levels EphrinBs are each composed of an ectodomain, a transmembrane domain and an intracellular domain; therefore, we analysed which ephrinB2 domains contribute to the loss of ephrinB2 in the absence of flotillin-1. We generated an ephrinB2 Δ60 mutant that has 60 amino acids deleted from the intracellular domain. Another mutant, ephrinB2 TM-Cyto , that lacks the ectodomain and consists of only the transmembrane and intracellular domains was also created, and was found to localize to the plasma membrane, similar to full-length ephrinB2 ( Supplementary Fig. 1c ). Injection of the F1aMO led to a significant decrease in protein abundance of the ephrinB2 Δ60 mutant, similar to the effect on wild-type ephrinB2 ( Fig. 3a ). In contrast, ephrinB2 TM-Cyto protein levels were unaffected by the F1aMO, indicating that the ephrinB2 ectodomain is an important determinant of ephrinB2 loss in the absence of flotillin-1 expression ( Fig. 3a ). 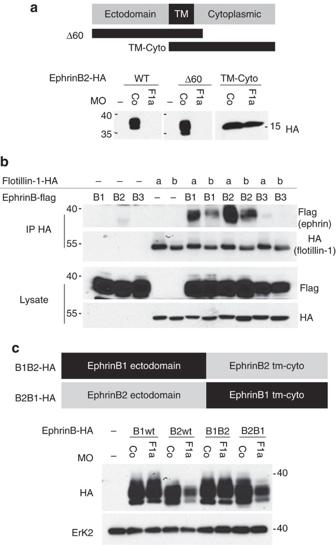Figure 3: The ephrinB2 ectodomain is important for decreased ephrinB2 expression in the absence of flotillin-1. (a) Deletion of the ephrinB2 ectodomain stabilizes its expression in the absence of flotillin-1. A schematic diagram of ephrinB2 and mutants is displayed, along with western blot analysis of embryos injected with CoMO or F1aMO and wild-type (WT) ephrinB2, ephrinB2Δ60or ephrinB2TM-CytoRNAs. (b) EphrinB1 as well as ephrinB2 are associated with flotillin-1. Flotillin-1a-HA or flotillin-1b-HA RNA was injected with or without ephrinB1-Flag, ephrinB2-Flag or ephrinB3-Flag RNA. Flotillin-1 was immunoprecipitated with anti-HA antibody, and immunoblotted with Flag antibody to detect ephrinBs. EphrinB1 and ephrinB2 were co-immunoprecipitated with flotillin-1a and flotillin-1b. Protein expression was confirmed in whole lysates by western blotting with the indicated antibodies. (c) The ephrinB2 ectodomain makes ephrinB2 protein susceptible to decreased expression in the presence of the F1aMO. The domain structure of B1B2-HA and B2B1-HA chimeric proteins is displayed, along with western blot analysis of embryos injected with F1aMO or CoMO and the indicated chimeric ephrinBs. Erk2 is used as a loading control. Figure 3: The ephrinB2 ectodomain is important for decreased ephrinB2 expression in the absence of flotillin-1. ( a ) Deletion of the ephrinB2 ectodomain stabilizes its expression in the absence of flotillin-1. A schematic diagram of ephrinB2 and mutants is displayed, along with western blot analysis of embryos injected with CoMO or F1aMO and wild-type (WT) ephrinB2, ephrinB2 Δ60 or ephrinB2 TM-Cyto RNAs. ( b ) EphrinB1 as well as ephrinB2 are associated with flotillin-1. Flotillin-1a-HA or flotillin-1b-HA RNA was injected with or without ephrinB1-Flag, ephrinB2-Flag or ephrinB3-Flag RNA. Flotillin-1 was immunoprecipitated with anti-HA antibody, and immunoblotted with Flag antibody to detect ephrinBs. EphrinB1 and ephrinB2 were co-immunoprecipitated with flotillin-1a and flotillin-1b. Protein expression was confirmed in whole lysates by western blotting with the indicated antibodies. ( c ) The ephrinB2 ectodomain makes ephrinB2 protein susceptible to decreased expression in the presence of the F1aMO. The domain structure of B1B2-HA and B2B1-HA chimeric proteins is displayed, along with western blot analysis of embryos injected with F1aMO or CoMO and the indicated chimeric ephrinBs. Erk2 is used as a loading control. Full size image Immunoprecipitation analysis shows that flotillin-1 interacts with both ephrinB1 and ephrinB2, but possesses much less affinity for ephrinB3 ( Fig. 3b ). Although ephrinB1 and ephrinB2 can both interact with flotillin-1, only ephrinB2 protein levels are compromised by flotillin-1 knockdown ( Fig. 2d,g ). Thus, we hypothesized that the ephrinB1 ectodomain may confer resistance to the effect of the F1aMO. To test this hypothesis, we made chimeric proteins composed of the ephrinB1 ectodomain and the ephrinB2 transmembrane and intracellular domains (B1B2-HA) or the ephrinB2 ectodomain and the ephrinB1 transmembrane and intracellular domains (B2B1-HA; Fig. 3c ). Consistent with our prediction, the B1B2-HA chimeric protein is stably expressed in F1aMO-injected embryos, while B2B1-HA expression is reduced in the presence of the F1aMO, similar to wild-type ephrinB2 ( Fig. 3c ). These data suggest that the reduction in ephrinB2 protein levels in the absence of flotillin-1 depends on the presence of the ephrinB2 ectodomain. ADAM10 leads to loss of ephrinB2 levels It has previously been shown that the ectodomain of ephrins can be cleaved by metalloproteases. For example, ephrinB1 is cleaved by matrix metalloproteinase-8 (MMP-8), and ephrin-A2 and ephrin-A5 are cleaved by ADAM10 (refs 7 , 10 , 21 ). Thus, we tested the possibility that a metalloprotease cleaves ephrinB2 and causes its decreased expression in the absence of flotillin-1. We found that two different broad-spectrum metalloprotease inhibitors, BB-94 and GM6001, both stabilized ephrinB2 expression in F1aMO-injected embryos ( Fig. 4a ). Recently, it was shown that Xenopus ephrinB1 and ephrinB2 are cleaved by ADAM13 (ref. 11 ). Among identified Xenopus orthologues of ADAM family proteins [22] , we selected ADAM10, ADAM13 and ADAM17 to test whether these ectodomain sheddases [22] , [23] , [24] , [25] may target ephrinB2 for cleavage and lead to the loss of its expression in the absence of flotillin-1. Surprisingly, knockdown of ADAM10 prevented a considerable portion of the loss of ephrinB2 protein that results from the introduction of the F1aMO, while knockdown of ADAM13 or ADAM17 had no such effect ( Fig. 4b,c ). Reintroduction of ADAM10 in the presence of the ADAM10 MO led to reduced ephrinB2 levels, supporting that ADAM10 specifically reduces ephrinB2 protein levels ( Fig. 4b ). Together, these data suggest that flotillin-1 inhibits ADAM10-mediated ephrinB2 loss. To confirm that ADAM10 is the specific metalloprotease that reduces ephrinB2 protein expression, ADAM10 and ADAM17 were overexpressed with ephrinB2 ( Fig. 4d ). Indeed, ADAM10 overexpression significantly lowers ephrinB2 protein levels in a dose-dependent manner, while ADAM17 has more subtle effects ( Fig. 4d ). To control for nonspecific competitive inhibition of ephrinB2 translation, GFP was overexpressed using the same RNA concentrations, and this had no effect on ephrinB2 protein levels ( Supplementary Fig. 2 ). 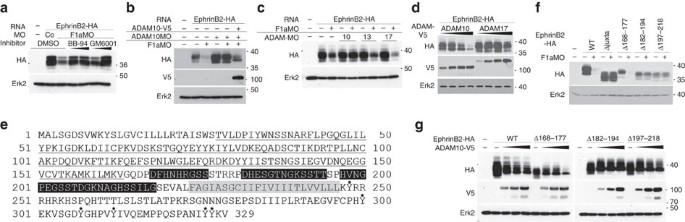Figure 4: ADAM10 is responsible for the loss of ephrinB2 expression in the absence of flotillin-1. (a) Metalloproteases are responsible for the loss of ephrinB2 expression in the absence of flotillin-1. Western blot analysis of ephrinB2-HA expression in the presence of CoMO or F1aMO and increasing amounts of the broad-spectrum metalloprotease inhibitors BB-94 and GM6001, as indicated. (b) ADAM10 reduces ephrinB2 expression, but is inhibited by the presence of endogenous flotillin-1. Western blot analysis of ephrinB2-HA in embryos injected with ADAM10 MO and/or F1aMO, and ADAM10-V5 RNA as indicated. Erk2 is used as a loading control. (c) Specific knockdown of ADAM10 rescues ephrinB2 loss in the presence of F1aMO. Western blot analysis of ephrinB2-HA in the presence of F1aMO alone or with the indicated ADAM MO. Erk2 is used as a loading control. (d) ADAM10 overexpression reduces ephrinB2 expression in a dose-dependent manner. Western blot analysis of embryos expressing ephrinB2-HA with increasing amounts of ADAM10-V5 or ADAM17-V5. (e) EphrinB2 amino-acid sequence. Black line indicates the globular region of the ephrinB2 ectodomain that is known to bind Eph receptors. The black boxes indicate amino acids 168–177, 182–194 and 197–218 in the juxtamembrane region of the ephrinB2 ectodomain, the grey box denotes the transmembrane domain and the six asterisks indicate the six tyrosine residues in the intracellular domain of ephrinB2. (f) Amino acids 182–214 of ephrinB2 are important for the decrease in ephrinB2 mediated by F1MO. Western blot analysis of ephrinB2 mutants lacking the indicated amino acids or juxtamembrane domain in the presence or absence of F1aMO. (g) Amino acids 182–214 of ephrinB2 are important for the decrease in ephrinB2 mediated by ADAM10. Western blot analysis of ephrinB2 mutants lacking the indicated amino acids or juxtamembrane domain in the presence or absence of ADAM10. Figure 4: ADAM10 is responsible for the loss of ephrinB2 expression in the absence of flotillin-1. ( a ) Metalloproteases are responsible for the loss of ephrinB2 expression in the absence of flotillin-1. Western blot analysis of ephrinB2-HA expression in the presence of CoMO or F1aMO and increasing amounts of the broad-spectrum metalloprotease inhibitors BB-94 and GM6001, as indicated. ( b ) ADAM10 reduces ephrinB2 expression, but is inhibited by the presence of endogenous flotillin-1. Western blot analysis of ephrinB2-HA in embryos injected with ADAM10 MO and/or F1aMO, and ADAM10-V5 RNA as indicated. Erk2 is used as a loading control. ( c ) Specific knockdown of ADAM10 rescues ephrinB2 loss in the presence of F1aMO. Western blot analysis of ephrinB2-HA in the presence of F1aMO alone or with the indicated ADAM MO. Erk2 is used as a loading control. ( d ) ADAM10 overexpression reduces ephrinB2 expression in a dose-dependent manner. Western blot analysis of embryos expressing ephrinB2-HA with increasing amounts of ADAM10-V5 or ADAM17-V5. ( e ) EphrinB2 amino-acid sequence. Black line indicates the globular region of the ephrinB2 ectodomain that is known to bind Eph receptors. The black boxes indicate amino acids 168–177, 182–194 and 197–218 in the juxtamembrane region of the ephrinB2 ectodomain, the grey box denotes the transmembrane domain and the six asterisks indicate the six tyrosine residues in the intracellular domain of ephrinB2. ( f ) Amino acids 182–214 of ephrinB2 are important for the decrease in ephrinB2 mediated by F1MO. Western blot analysis of ephrinB2 mutants lacking the indicated amino acids or juxtamembrane domain in the presence or absence of F1aMO. ( g ) Amino acids 182–214 of ephrinB2 are important for the decrease in ephrinB2 mediated by ADAM10. Western blot analysis of ephrinB2 mutants lacking the indicated amino acids or juxtamembrane domain in the presence or absence of ADAM10. Full size image Since ADAM10 cleaves the juxtamembrane region of ephrin-A2 (ref. 7 ), and MMP-8 cleaves the juxtamembrane region of ephrinB1 (ref. 20 ), we tested whether this region of the ephrinB2 ectodomain is important for loss of ephrinB2 expression in the absence of flotillin-1 ( Fig. 4e ). Indeed, juxtamembrane deletion mutants were stably expressed in the presence of F1aMO ( Fig. 4e,f ), and specifically deleting sequences in this region (amino acids 182–194 and 197–218) renders ephrinB2 resistant to the ADAM10-mediated effect ( Fig. 4g ). These data suggest that ADAM10 cleaves the juxtamembrane region of the ephrinB2 ectodomain. ADAM10 cleaves ephrinB2 and regulates ephrinB2 protein levels ADAM10 cleavage of ephrinB2 should result in two fragments: a 25-kDa amino-terminal fragment and a 15-kDa carboxyl-terminal fragment (CTF). Without any treatment, the ~40-kDa full-length ephrinB2-HA protein and two ephrinB2 CTF bands of ~15 kDa were detected in embryonic lysates, suggesting that ephrinB2 is cleaved by endogenous ADAM10 and further processed ( Fig. 5a ). Since it is known that MMP-8 can cleave the ephrinB1 ectodomain and that subsequently γ-secretase cleaves the juxtamembrane region of the intracellular domain [20] , we speculated that γ-secretase may also cleave the ephrinB2 intracellular domain. This could produce the two observed CTF bands: an upper band generated by ADAM10 cleavage, and a lower band resulting from both ADAM10 and γ-secretase cleavage. When ADAM10 was overexpressed, full-length ephrinB2 was reduced and the upper CTF band was increased, indicating that ADAM10 indeed cleaves ephrinB2 and reduces its expression ( Fig. 5a ). Conversely, when embryos were treated with the ADAM10-specific inhibitor GI254023X, full-length ephrinB2 was slightly increased and the upper CTF band was reduced, with the greatest difference detected in the embryos overexpressing ADAM10 ( Fig. 5a ). In addition, we used co-expression and co-IP analysis in embryos to determine whether ADAM10 associates with ephrinB2. We found that ephrinB2 is robustly present in ADAM10 immune complexes, but found at relatively low levels in ADAM17 immmune complexes, supporting the idea that ephrinB2 is specifically cleaved by the ADAM10 metalloprotease ( Fig. 5b ). Moreover, although ephrinB1 also associates with ADAM10 in co-IPs from Xenopus oocytes co-expressing both proteins ( Fig. 5c ), only ephrinB2 is a target of ADAM10 cleavage in a dose-dependent manner in embryos ( Fig. 5d ). In HT-29 cells, endogenous ADAM10 was co-IP'd in ephrinB2 immune complexes ( Fig. 5e ), confirming that ephrinB2 and ADAM10 associate either directly or indirectly in vivo . 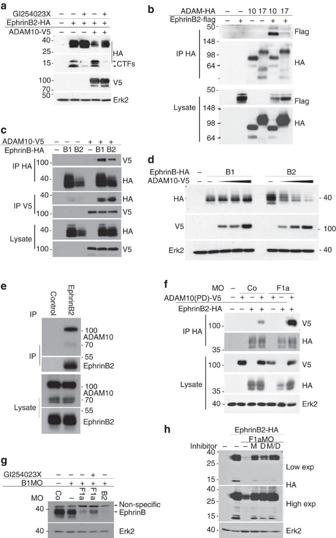Figure 5: ADAM10 cleaves ephrinB2 and regulates ephrinB2 protein levels. (a) ADAM10 is responsible for shedding of the ephrinB2 ectodomain. Western blot analysis of embryos expressing ephrinB2-HA with ADAM10-V5 and/or the ADAM10-specific inhibitor GI254023X. The full-length ephrinB2-HA and the C-terminal fragments (CTFs) of ephrinB2-HA are indicated. ADAM10-V5 is indicated, as is the Erk2 loading control. (b) EphrinB2 associates with ADAM10. ADAM10-HA immunoprecipitation and western blot analysis from embryonic lysates co-expressing ephrinB2-Flag and ADAM10-HA or ADAM17-HA. Direct lysates are probed with anti-Flag or HA as indicated. (c) ADAM10 associates with ephrinB1 as well as ephrinB2. Western blot analysis of the indicated IPs or direct lysates from oocytes expressing ephrinB2-HA or ephrinB1-HA alone or with ADAM10-V5. (d) ADAM10 specifically targets ephrinB2. Western blot analysis with indicated antibodies of lysates from embryos exogenously expressing increasing amounts of ADAM10-V5 along with ephrinB1-HA or ephrinB2-HA. (e) Endogenous ADAM10 associates with ephrinB2. EphrinB2 was immunoprecipitated from HT-29 cells and western blot analysis was performed using anti-ephrinB2 or ADAM10 antibodies. EphrinB2 and ADAM10 expression levels in HT-29 cell lysates are shown. (f) In the presence of MG132, F1aMO leads to increased association between exogenously expressed ephrinB2 and ADAM10. Western blot analysis of the HA (ephrinB2) IPs and direct lysates from embryos co-expressing ephrinB2-HA and an ADAM10 mutant with compromised protease activity (ADAM10 PD-V5) and injected with the indicated MOs. (g) Endogenous ephrinB2 is cleaved and degraded in the presence of F1aMO, but is partially rescued by an ADAM10-specific inhibitor. Western blot analysis of lysates from neural folds of embryos injected with the indicated MOs, and the ADAM10 inhibitor GI254023X (stage 9 injections into the blastocoel). Western blots were probed using C-18 (pan-ephrinB) and ERK2 antibodies. (h) EphrinB2 is degraded by both the proteosomal and dynamin-dependent degradation pathways in the absence of flotillin-1. Western blot analysis with the indicated antibodies of embryos injected with ephrinB2-HA RNA alone or with F1aMO, and treated with vehicle control dimethylsulphoxide (−), or MG132 (M), and/or dynamin inhibitor dynasore (D). Erk2 is used as a loading control. Figure 5: ADAM10 cleaves ephrinB2 and regulates ephrinB2 protein levels. ( a ) ADAM10 is responsible for shedding of the ephrinB2 ectodomain. Western blot analysis of embryos expressing ephrinB2-HA with ADAM10-V5 and/or the ADAM10-specific inhibitor GI254023X. The full-length ephrinB2-HA and the C-terminal fragments (CTFs) of ephrinB2-HA are indicated. ADAM10-V5 is indicated, as is the Erk2 loading control. ( b ) EphrinB2 associates with ADAM10. ADAM10-HA immunoprecipitation and western blot analysis from embryonic lysates co-expressing ephrinB2-Flag and ADAM10-HA or ADAM17-HA. Direct lysates are probed with anti-Flag or HA as indicated. ( c ) ADAM10 associates with ephrinB1 as well as ephrinB2. Western blot analysis of the indicated IPs or direct lysates from oocytes expressing ephrinB2-HA or ephrinB1-HA alone or with ADAM10-V5. ( d ) ADAM10 specifically targets ephrinB2. Western blot analysis with indicated antibodies of lysates from embryos exogenously expressing increasing amounts of ADAM10-V5 along with ephrinB1-HA or ephrinB2-HA. ( e ) Endogenous ADAM10 associates with ephrinB2. EphrinB2 was immunoprecipitated from HT-29 cells and western blot analysis was performed using anti-ephrinB2 or ADAM10 antibodies. EphrinB2 and ADAM10 expression levels in HT-29 cell lysates are shown. ( f ) In the presence of MG132, F1aMO leads to increased association between exogenously expressed ephrinB2 and ADAM10. Western blot analysis of the HA (ephrinB2) IPs and direct lysates from embryos co-expressing ephrinB2-HA and an ADAM10 mutant with compromised protease activity (ADAM10 PD-V5) and injected with the indicated MOs. ( g ) Endogenous ephrinB2 is cleaved and degraded in the presence of F1aMO, but is partially rescued by an ADAM10-specific inhibitor. Western blot analysis of lysates from neural folds of embryos injected with the indicated MOs, and the ADAM10 inhibitor GI254023X (stage 9 injections into the blastocoel). Western blots were probed using C-18 (pan-ephrinB) and ERK2 antibodies. ( h ) EphrinB2 is degraded by both the proteosomal and dynamin-dependent degradation pathways in the absence of flotillin-1. Western blot analysis with the indicated antibodies of embryos injected with ephrinB2-HA RNA alone or with F1aMO, and treated with vehicle control dimethylsulphoxide (−), or MG132 (M), and/or dynamin inhibitor dynasore (D). Erk2 is used as a loading control. Full size image Having established that ADAM10 can associate with ephrinB2, we considered whether flotillin-1 may, in part, prevent ADAM10 cleavage by restricting the interaction between these two proteins. To address this possibility, we co-expressed ephrinB2 and an ADAM10 point mutant with compromised protease activity (to prevent cleavage of ephrinB2) in Xenopus embryos in the presence of the proteasomal inhibitor MG132 and the F1MO or CoMO. Co-IP analysis shows a marked increase in the ADAM10 mutant detected in ephrinB2 immune complexes from the embryos with flotillin-1 knocked down when compared with those with control MO ( Fig. 5f ). This result suggests that flotillin-1, at least in part, inhibits the association between ephrinB2 and ADAM10 in vivo . To confirm that endogenous ephrinB2 is targeted by ADAM10, embryos were injected with B1MO alone or with F1aMO in either the absence or presence of the ADAM10-specific inhibitor. The dorsal axial region (neural fold) was excised and subjected to western blot analysis using the ephrinB antibody. In the absence of ephrinB1, ephrinB2 levels are detected in the dorsal axial region with this antibody. As expected, the introduction of an F1aMO results in a dramatic reduction in ephrinB2 protein levels, and this is partially rescued by treatment with the ADAM10-specific inhibitor ( Fig. 5g ). Since the F1MO-mediated decrease in ephrinB2 is quite robust ( Fig. 5a,g ), we examined whether there was additional processing via proteasomal or lysosomal degradation as well as the ADAM10-mediated cleavage that would be expected to remove cell surface ephrinB2. Inhibitors of proteasomal degradation (MG132), or dynamin-dependent endocytosis (dynasore) were used to determine the effective pathways employed in response to F1MO-induced regulation of ephrinB2 protein levels. Xenopus embryos were cultured until the neurula stage after the introduction of HA-tagged ephrinB2 RNA alone or along with F1aMO. These embryos were cultured in the inhibitors for 5 h, and then western blot analysis was performed. As expected, flotillin-1 knockdown resulted in a dramatic loss of ephrinB2 protein in the embryonic lysates ( Fig. 5h ). Treatment with both MG132 and dynasore efficiently rescued ephrinB2 levels, while dynasore alone increased ephrinB2 levels, but to a lesser degree than MG132 alone ( Fig. 5h ). Of note, the CTFs are similarly affected by these reagents ( Fig. 5h ). These data indicate that in the absence of flotillin-1, full-length ephrinB2 and the ADAM10-cleaved CTFs are targeted for destruction through the lysosomal and proteasomal pathways. We also examined whether the observed F1aMO-mediated reduction in ephrinB2 protein was due to a decrease in the half-life of ephrinB2 (as would be expected if the protein is being degraded), and whether cleavage by ADAM10 promotes this activity. For this purpose, we carefully titrated the amount of injected ephrinB2 RNA along with CoMO or F1aMO to yield roughly equivalent ephrinB2 protein levels when embryos reached the neurula stage. The embryos were then injected with cycloheximide (CHX) or with both CHX and ADAM10 inhibitor, and cultured in CHX to block further protein synthesis for 5 h ( Fig. 6a,b ). Western blot analysis shows that ephrinB2 levels are reduced by half within 153 min (~2.5 h) after the addition of CHX to control MO-containing embryos. In the F1aMO-containing embryos, the half-life of ephrinB2 is reduced to 57 min (~1 h; Fig. 6a,b ). In contrast, the half-life of ephrinB2 is actually extended to 102 min (~1.7 h) in the F1aMO plus ADAM10 inhibitor-injected embryos ( Fig. 6a,b ). These data are consistent with flotillin-1 hindering ephrinB2 degradation, in part, by inhibiting its cleavage by ADAM10. 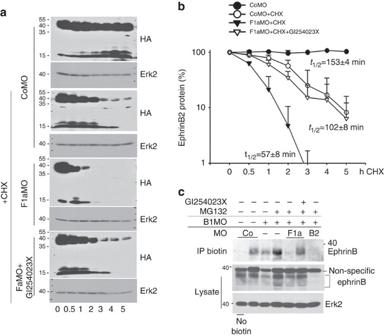Figure 6: EphrinB2 protein half-life is decreased in the absence of flotillin-1 and partially rescued by the ADAM10 inhibitor. (a) Two-cell-stage embryos were injected with carefully titratedephrinB2-HARNA along with control MO or F1aMO to yield roughly equivalent ephrinB2 protein levels when embryos reached the early neurula stages. A group of the injected embryos was subjected to a secondary injection into the blastocoel at stage 9 with ADAM10 inhibitor (10 nl of 1 mM), and the archenteron cavity (stage 14) with CHX (10 nl of 75 μg μl−1), and externally incubated in CHX (7.5 μg μl−1) to block further protein synthesis for the indicated times. Western blot analysis was performed on the embryonic lysates using HA antibodies or Erk2 antibodies (as a loading control). (b) A graph of the mean band intensities as measured by Image J software shows the approximate half-lives in the presence of CHX and the indicated MOs and ADAM10 inhibitor. The ephrinB2 C-terminal fragments (short arrow) and the full-length protein (long arrow) are indicated. These data are the result of three independent experiments and ± represents s.d. (c) Endogenous surface ephrinB2 levels are reduced by knockdown of flotillin-1, but prominently rescued by the ADAM10 inhibitor. Embryos were injected with the indicated MOs and inhibitors. Neural folds were excised and left non-biotinylated (lane 1) or biotinylated. Lysates were prepared and cell surface proteins immunoprecipitated with streptavidin-conjugated sepharose. Western blot analysis of biotin-labelled cell surface proteins was performed using anti-ephrinB antibody. Direct western blot analysis of neural fold lysates were probed for ephrinB. Erk2 expression is shown as a loading control. Figure 6: EphrinB2 protein half-life is decreased in the absence of flotillin-1 and partially rescued by the ADAM10 inhibitor. ( a ) Two-cell-stage embryos were injected with carefully titrated ephrinB2-HA RNA along with control MO or F1aMO to yield roughly equivalent ephrinB2 protein levels when embryos reached the early neurula stages. A group of the injected embryos was subjected to a secondary injection into the blastocoel at stage 9 with ADAM10 inhibitor (10 nl of 1 mM), and the archenteron cavity (stage 14) with CHX (10 nl of 75 μg μl −1 ), and externally incubated in CHX (7.5 μg μl −1 ) to block further protein synthesis for the indicated times. Western blot analysis was performed on the embryonic lysates using HA antibodies or Erk2 antibodies (as a loading control). ( b ) A graph of the mean band intensities as measured by Image J software shows the approximate half-lives in the presence of CHX and the indicated MOs and ADAM10 inhibitor. The ephrinB2 C-terminal fragments (short arrow) and the full-length protein (long arrow) are indicated. These data are the result of three independent experiments and ± represents s.d. ( c ) Endogenous surface ephrinB2 levels are reduced by knockdown of flotillin-1, but prominently rescued by the ADAM10 inhibitor. Embryos were injected with the indicated MOs and inhibitors. Neural folds were excised and left non-biotinylated (lane 1) or biotinylated. Lysates were prepared and cell surface proteins immunoprecipitated with streptavidin-conjugated sepharose. Western blot analysis of biotin-labelled cell surface proteins was performed using anti-ephrinB antibody. Direct western blot analysis of neural fold lysates were probed for ephrinB. Erk2 expression is shown as a loading control. Full size image Since flotillin-1 is known to affect trafficking of some transmembrane proteins [26] , we examined whether the reduction in the endogenous ephrinB2 protein in the absence of flotillin-1 is similarly affected at the cell surface when protein degradation is blocked. Xenopus embryos were injected with B1MO and treated with MG132 to prevent ephrinB2 degradation. A group of these embryos was also injected with F1aMO in the presence or absence of the ADAM10-specific inhibitor that prevents cleavage and thus loss from the cell surface. The dorsal axial region was excised at stage 16–18 and the cell surface proteins were biotinylated. Immunoprecipitation of cell surface proteins from lysates of the explants was performed using streptavidin-conjugated sepharose, and western blotting with ephrinB antibody. As expected, use of both B1MO and B2MO removes nearly all the detectable ephrinBs in the dorsal axial region ( Fig. 6c ). In the presence of MG132, the F1aMO causes a prominent reduction in biotinylated (cell surface) ephrinB2 protein, and this is partially, but considerably rescued in the presence of the ADAM10 inhibitor ( Fig. 6c ). These data indicate that loss of flotillin-1 considerably reduces endogenous cell surface ephrinB2 protein levels by promoting ADAM10-mediated cleavage. EphrinB2 and flotillin-1 morphants show neural tube defects To assess whether there is a functional effect mediated by the interaction between flotillin-1 and ephrinB2, we examined the effect of knocking down ephrinB2 in Xenopus embryos, which express ephrinB2 at early stages of neural tube formation. When embryos were injected with the B2MO, only 10.2% displayed a closed neural tube by stage 18/19 ( Fig. 7a,b ), while 96.5% of the CoMO-injected embryos had closed neural tubes ( Fig. 7a,b ). At later stages, profound delays or failure of neural tube closure were observed ( Fig. 7c,d ). This effect is specific to the B2MO, since MO-mediated knockdown of ephrinB1 did not disrupt neural tube closure ( Fig. 7e ). Further evidence of the specificity of the B2MO and the requirement for ephrinB2 in neural tube closure is provided by the rescue of neural tube defects (59.6% closed neural tubes) by re-expressing ephrinB2 using B2 11MT RNA, which is resistant to the B2MO ( Fig. 7a,b ). 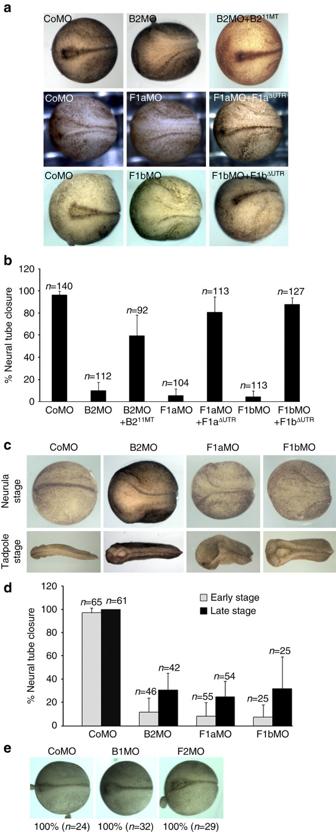Figure 7: EphrinB2 and flotillin-1 morphants show neural tube closure defects. (a) Neural tube closure defects in ephrinB2 or flotillin-1 morphants. Dorsal view of stage 18 control, ephrinB2, flotillin-1a or flotillin-1b MO-injected embryos, and those co-injected with morpholino-resistant RNA (B211MT-HA for B2MO, F1aΔUTR-Flag for F1aMO and F1bΔUTR-Flag for F1bMO); left is anterior and right is posterior. (b) Quantification of neural tube closure defects in ephrinB2 or flotillin-1 morphants. Embryos showing a single dorsal line were counted as having closed neural tubes. At least three independent experiments were performed and error bars indicate s.d. (c) B2MO, F1aMO, or F1bMO were injected into embryos, and neural tube closure was examined at neurula (stage 18/19) and swimming tadpole stages. Note the anterior neural tube defects. (d) Percentage of neural tube closure in B2MO-, F1aMO-, or F1bMO-injected embryos. Note that the percentage of neural tube closure is somewhat elevated at later stages in B2MO-, F1aMO- and F1bMO-injected embryos, indicating that some of the embryos displayed a profound delay in neural tube closure, while others retain an open neural tube. Error bars indicate s.d. (e) EphrinB1- MO- or flotillin-2 MO-injected embryos show normal neural tube closure. Figure 7: EphrinB2 and flotillin-1 morphants show neural tube closure defects. ( a ) Neural tube closure defects in ephrinB2 or flotillin-1 morphants. Dorsal view of stage 18 control, ephrinB2, flotillin-1a or flotillin-1b MO-injected embryos, and those co-injected with morpholino-resistant RNA (B2 11MT -HA for B2MO, F1a ΔUTR -Flag for F1aMO and F1b ΔUTR -Flag for F1bMO); left is anterior and right is posterior. ( b ) Quantification of neural tube closure defects in ephrinB2 or flotillin-1 morphants. Embryos showing a single dorsal line were counted as having closed neural tubes. At least three independent experiments were performed and error bars indicate s.d. ( c ) B2MO, F1aMO, or F1bMO were injected into embryos, and neural tube closure was examined at neurula (stage 18/19) and swimming tadpole stages. Note the anterior neural tube defects. ( d ) Percentage of neural tube closure in B2MO-, F1aMO-, or F1bMO-injected embryos. Note that the percentage of neural tube closure is somewhat elevated at later stages in B2MO-, F1aMO- and F1bMO-injected embryos, indicating that some of the embryos displayed a profound delay in neural tube closure, while others retain an open neural tube. Error bars indicate s.d. ( e ) EphrinB1- MO- or flotillin-2 MO-injected embryos show normal neural tube closure. Full size image Having established that knockdown of flotillin-1 in embryos leads to a dramatic reduction in ephrinB2 protein levels that is at least partly dependent on cleavage via ADAM10, we decided to test whether knockdown of flotillin-1 also affected neural tube closure. Both F1aMO and F1bMO caused neural tube closure defects that are similar to ephrinB2 morphant phenotypes ( Fig. 7a,b ). Only 5.7 and 4.6% of F1aMO- or F1bMO-injected stage 18/19 embryos displayed closed neural tubes, while flotillin-2 morphants showed normal neural tube closure ( Fig. 7e ). Importantly, these defects were rescued by exogenous flotillin-1a or -1b expression (81.0% by F1a ΔUTR -Flag and 87.7% by F1b ΔUTR -Flag, respectively). To test whether there was redundancy between the a and b paralogues of flotillin-1, RNA encoding either paralogue was expressed along with exogenous ephrinB2 in F1aMO-injected embryos. Western analysis shows that each paralogue can rescue ephrinB2 protein levels in the embryos injected with F1aMO ( Supplementary Fig. 3a ), and a partial, but sizeable rescue of neural tube closure is observed ( Supplementary Fig. 3b ) and evidenced by a clear reduction in the gap width between the neural folds ( Supplementary Fig. 3c ). These data suggest that the isoforms have at least partially overlapping functions. Neural tube formation is a complex process [27] that transforms a flat oval sheet of thickened epithelium (the neural plate) into a neural tube. This process is driven by three overlapping events. First, convergence and extension movements elongate the neural plate [28] . Second, apical constriction of the neuroepithelial cells within the neural plate brings the sides of the plate closer together. Third, the lateral edges of the plate elevate to make neural folds. The neural folds move towards the dorsal midline, where they meet and fuse to form a tubular structure, finalizing the separation between the future epidermis and the neural epithelium. Flotillin-1 and ephrinB2 morphants fail to apically constrict CoMO-injected embryos and B2MO- or F1MO-injected embryos appear to form normal neural plates until stage 14. Strikingly, after this stage we observed that ephrinB2 and flotillin-1 morphants develop broad neural grooves and lack elevated neural folds ( Fig. 7a–d ), indicating a possible problem in the process of neural plate bending, which is driven by apical constriction [29] . When one side of the embryo is injected with B2MO or F1bMO, it displays apical constriction defects of the neuroepithelium, while the uninjected side retains normal morphology and wedge-shaped cells ( Fig. 8a ). Cell lengths are significantly decreased and cell widths are increased on the B2MO- or F1bMO-injected side when compared with the uninjected side. The average ratio of the length of the apical surface to the cell perimeter was calculated using five different cells adjacent to the midline. The ratio increased for cells harbouring the B2MO or the F1bMO compared with uninjected cells ( Fig. 8b ), indicating that loss of ephrinB2 or flotillin-1b reduces apical constriction in the neuroepithelium. 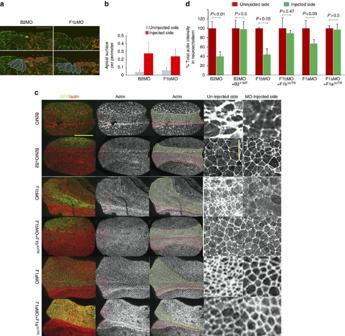Figure 8: Neuroepithelial cells of flotillin-1 and ephrinB2 morphants fail to apically constrict in the presumptive neural tube. (a) Apical constriction defects of ephrinB2 and flotillin-1 morphants. B2MO or F1bMO were injected into one side of the embryos along with GFP RNA as a tracer. At the neurula stage, embryos were stained with anti-tubulin (green) antibody to outline the cells and with anti-GFP (red) antibody to label the injected side. Cell shapes are outlined below. Blue, uninjected cells; red, MO-injected cells. Scale bar, 50 μm. (b) The average ratios of the apical surfaces to the perimeters among five different cells on each side of the midline were calculated for five different embryos. Blue bars, uninjected side; red bars, MO-injected side. (c) Decreased actin intensity in ephrinB2 or flotillin-1 morphants. Each embryo was injected with the indicated MO and GFP RNA with or without the appropriate rescue RNA as indicated. GFP (green) shows the injected side and actin is stained red (phalloidin staining). In the third column, the neuroepithelium is outlined in green on the MO-injected side and red on the uninjected side. Red boxed regions from embryos in the second column are presented as enlarged images in the fourth and fifth columns. Scale bar, 300 μm (horizontal); 50 μm (vertical). (d) Total actin intensity is decreased in ephrinB2 or flotillin-1 morphants. Percent total actin intensities were calculated for the uninjected or injected side of the embryo using the methodology described in the Methods section. A two-tailedt-test was used to generate thePvalue. These results represent three independent experiments. Error bars represent s.d. Figure 8: Neuroepithelial cells of flotillin-1 and ephrinB2 morphants fail to apically constrict in the presumptive neural tube. ( a ) Apical constriction defects of ephrinB2 and flotillin-1 morphants. B2MO or F1bMO were injected into one side of the embryos along with GFP RNA as a tracer. At the neurula stage, embryos were stained with anti-tubulin (green) antibody to outline the cells and with anti-GFP (red) antibody to label the injected side. Cell shapes are outlined below. Blue, uninjected cells; red, MO-injected cells. Scale bar, 50 μm. ( b ) The average ratios of the apical surfaces to the perimeters among five different cells on each side of the midline were calculated for five different embryos. Blue bars, uninjected side; red bars, MO-injected side. ( c ) Decreased actin intensity in ephrinB2 or flotillin-1 morphants. Each embryo was injected with the indicated MO and GFP RNA with or without the appropriate rescue RNA as indicated. GFP (green) shows the injected side and actin is stained red (phalloidin staining). In the third column, the neuroepithelium is outlined in green on the MO-injected side and red on the uninjected side. Red boxed regions from embryos in the second column are presented as enlarged images in the fourth and fifth columns. Scale bar, 300 μm (horizontal); 50 μm (vertical). ( d ) Total actin intensity is decreased in ephrinB2 or flotillin-1 morphants. Percent total actin intensities were calculated for the uninjected or injected side of the embryo using the methodology described in the Methods section. A two-tailed t -test was used to generate the P value. These results represent three independent experiments. Error bars represent s.d. Full size image Apical constriction results from the contraction of apically localized filamentous actin (F-actin), driven by the motor protein myosin [28] , [29] . Therefore, we examined F-actin intensities in neuroepithelium in the presence or absence of ephrinB2 or flotillin-1. B2MO, F1aMO or F1bMO was injected along with GFP RNA (as a tracer) into one side of the embryos, and Texas-Red-conjugated phalloidin staining was performed to compare F-actin levels on the uninjected control side with those on the MO-injected side. Injection of each MO (B2MO, F1aMO or F1bMO) caused a broadening of the neural plate and a significant decrease in total actin intensity in the neural fold ( Fig. 8c,d ). The decrease in intensity within individual cells can also be observed ( Fig. 8c , insets). The B2MO as well as the F1aMO or F1bMO notably reduced the total actin intensity when compared to the uninjected control side of the neural plate ( Fig. 8d ). This B2MO- or F1MO-mediated decrease in F-actin intensity levels can be rescued by the introduction of B2 11MT -HA or F1 ΔUTR -Flag RNAs, respectively. These data are reflective and consistent with the experiments showing that the apical surface of the neural fold cells are increased ( Fig. 8a,b ). We found that neither ephrinB2 nor flotillin-1 overexpression was capable of inducing apical constriction in naive ectodermal explants as evidenced by actin staining or membrane-bound GFP visualization ( Supplementary Fig. 4 ). Taken together, these data indicate that ephrinB2 and flotillin-1 are required for a normal actin cytoskeleton in neuroepithelial cells, and the loss of either protein leads to failure of apical constriction. To test whether the defects in neural tube closure observed in flotillin-1 morphants can be attributed to ephrinB2 loss, we elevated ephrinB2 expression in F1aMO-injected embryos by using a 10-fold greater amount of ephrinB2 RNA than that required for rescue of a B2MO phenotype ( Fig. 9a,b ). Interestingly, elevating ephrinB2 expression in F1aMO-injected embryos partially rescued the neural tube closure defects ( Fig. 9a–c ). EphrinB2-HA expression in F1aMO-injected embryos was confirmed by western blot analysis ( Fig. 9b ). Consistent with this rescue, sufficient expression of ephrinB2-HA (1.5 ng of RNA) in the presence of the F1aMO elevated the total actin intensity in the neuroepithelium to near normal levels, while insufficient expression of ephrinB2-HA (1 ng of RNA) in F1aMO-injected embryos still caused a decrease in total actin intensity to about 56% of that of the uninjected control side ( Fig. 9d–f ). Taken together, these results suggest that flotillin-1 maintains ephrinB2 expression and neural tube closure, in part, by reducing the susceptibility of ephrinB2 to ADAM10-mediated cleavage. 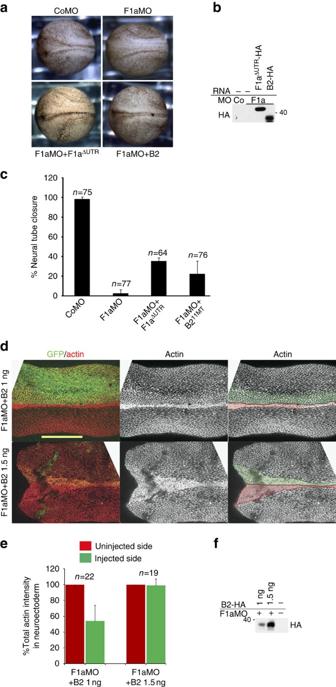Figure 9: Neural tube closure defects of F1aMO-injected embryos are caused by loss of ephrinB2. (a) EphrinB2 expression in F1aMO-injected embryos rescues neural tube closure defects. Dorsal view of embryos injected with F1aMO or CoMO alone or with F1aΔUTR-HA or ephrinB2-HA (1.5 ng) RNA as indicated. (b) Titration of ephrinB2-HA expression with F1aMO. Western blot analysis of embryos fromainjected with F1aMO and ephrinB2-HA RNA (1.5 ng) or F1aΔUTR-HA RNA. (c) EphrinB2-HA expression as well as flotillin-1aΔUTR-HA expression partially rescues neural tube closure defects observed in F1aMO-injected embryos. Percentages of neural tube closures inawere calculated for the indicated MO and RNA injections. The results represent three independent experiments. Error bars represent s.d. (d) F1aMO-induced decrease in mean actin intensity is rescued by ephrinB2. Confocal image of the neural tube of embryos injected with a high level (1.5 ng) or a low level (1 ng) of ephrinB2 RNA and the F1aMO. GFP (green) marks the injected side and actin is stained red (phalloidin staining) on both sides as inFig. 8c. Scale bar, 300 μm. (e) Quantification of total actin intensity in neuroepithelium fromd. These results represent two independent experiments. Error bars denote s.d. (f) Western blot showing ephrinB2 expression levels ind. Figure 9: Neural tube closure defects of F1aMO-injected embryos are caused by loss of ephrinB2. ( a ) EphrinB2 expression in F1aMO-injected embryos rescues neural tube closure defects. Dorsal view of embryos injected with F1aMO or CoMO alone or with F1a ΔUTR -HA or ephrinB2-HA (1.5 ng) RNA as indicated. ( b ) Titration of ephrinB2-HA expression with F1aMO. Western blot analysis of embryos from a injected with F1aMO and ephrinB2-HA RNA (1.5 ng) or F1a ΔUTR -HA RNA. ( c ) EphrinB2-HA expression as well as flotillin-1a ΔUTR -HA expression partially rescues neural tube closure defects observed in F1aMO-injected embryos. Percentages of neural tube closures in a were calculated for the indicated MO and RNA injections. The results represent three independent experiments. Error bars represent s.d. ( d ) F1aMO-induced decrease in mean actin intensity is rescued by ephrinB2. Confocal image of the neural tube of embryos injected with a high level (1.5 ng) or a low level (1 ng) of ephrinB2 RNA and the F1aMO. GFP (green) marks the injected side and actin is stained red (phalloidin staining) on both sides as in Fig. 8c . Scale bar, 300 μm. ( e ) Quantification of total actin intensity in neuroepithelium from d . These results represent two independent experiments. Error bars denote s.d. ( f ) Western blot showing ephrinB2 expression levels in d . Full size image Loss of ADAM10 rescues F1aMO-induced neural tube defects One prediction from this model is that the neural tube closure defect induced by loss of flotillin-1 may be rescued by the disruption of ADAM10 function. To test this prediction, embryos were injected with either F1aMO or ADAM10 MO alone or together, and the gap width of the neural tube at stage 18 was examined. ADAM10 MO substantially rescued the neural tube closure defect induced by F1aMO, as evidenced by the morphology and the reduction in gap width between the neural folds ( Fig. 10a,b ). The reciprocal experiment also supports this concept. Introduction of ADAM10 RNA into two dorsal blastomeres of four-cell-stage embryos cause a neural tube closure defect later in development, while the control ADAM10 construct having compromised metalloprotease activity fails to cause this defect ( Fig. 10c–e ). 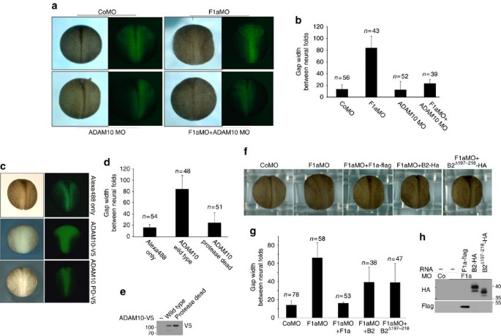Figure 10: Loss of ADAM10 rescues F1aMO-induced neural tube defects, while overexpression of ADAM10 causes neural tube defects. (a) Knockdown of ADAM10 rescues neural tube closure defects induced by F1aMO. Two dorsal cells of four-cell-stage embryos were injected with Alexa 488-conjugated dextran (green) and the F1aMO alone or an ADAM10 MO, or both. Presented are dorsal view images with light and fluorescent microscopy. (b) The gap width of the neural tubes in the embryos injected with the indicated MOs inawere measured and the average gap width and s.d. are presented in the histogram. (c) Overexpression of ADAM10 causes neural tube closure defects. Dorsal view with light and fluorescent microscopy of embryos that were injected with Alexa 488-conjugated dextran (green—tracer) alone, or with ADAM10-V5 RNA or RNA encoding an ADAM10 mutant with compromised protease activity (ADAM10 PD-V5). (d) The width of the neural tubes in the embryos injected with the indicated reagents incwere measured and the average width and s.d. are presented in the histogram. (e) Western blot of lysates from the injected embryos inc, probed with V5 antibody. (f) An ephrinB2 mutant that is resistant to ADAM10 cleavage rescues F1aMO-induced neural tube defects. Dorsal view of embryos that were injected with either control MO or F1aMO and RNA encoding flotillin-1a-Flag, or high levels of ephrinB2-HA (1.6 ng per embryo), or low levels of cleavage-resistant ephrinB2Δ197-218-HA (0.4 ng per embryo). (g) The gap widths of the neural tubes in the embryos injected with the indicated reagents infwere measured and the average width and s.d. are presented in the histogram. (h) Western blot analysis of the embryonic lysates fromfusing the indicated antibodies to show expression of flotillin-1-Flag, ephrinB2-HA and ephrinB2Δ197-218. Figure 10: Loss of ADAM10 rescues F1aMO-induced neural tube defects, while overexpression of ADAM10 causes neural tube defects. ( a ) Knockdown of ADAM10 rescues neural tube closure defects induced by F1aMO. Two dorsal cells of four-cell-stage embryos were injected with Alexa 488-conjugated dextran (green) and the F1aMO alone or an ADAM10 MO, or both. Presented are dorsal view images with light and fluorescent microscopy. ( b ) The gap width of the neural tubes in the embryos injected with the indicated MOs in a were measured and the average gap width and s.d. are presented in the histogram. ( c ) Overexpression of ADAM10 causes neural tube closure defects. Dorsal view with light and fluorescent microscopy of embryos that were injected with Alexa 488-conjugated dextran (green—tracer) alone, or with ADAM10-V5 RNA or RNA encoding an ADAM10 mutant with compromised protease activity (ADAM10 PD-V5). ( d ) The width of the neural tubes in the embryos injected with the indicated reagents in c were measured and the average width and s.d. are presented in the histogram. ( e ) Western blot of lysates from the injected embryos in c , probed with V5 antibody. ( f ) An ephrinB2 mutant that is resistant to ADAM10 cleavage rescues F1aMO-induced neural tube defects. Dorsal view of embryos that were injected with either control MO or F1aMO and RNA encoding flotillin-1a-Flag, or high levels of ephrinB2-HA (1.6 ng per embryo), or low levels of cleavage-resistant ephrinB2 Δ197-218 -HA (0.4 ng per embryo). ( g ) The gap widths of the neural tubes in the embryos injected with the indicated reagents in f were measured and the average width and s.d. are presented in the histogram. ( h ) Western blot analysis of the embryonic lysates from f using the indicated antibodies to show expression of flotillin-1-Flag, ephrinB2-HA and ephrinB2 Δ197-218 . Full size image Finally, expression of the ephrinB2 Δ197-218 mutant that is resistant to ADAM10 cleavage partially rescues neural tube closure in F1aMO-injected embryos ( Fig. 10f–h ). This cleavage-resistant mutant RNA rescues neural tube closure at levels fourfold below the amount required for an equivalent rescue using wild-type ephrinB2 RNA ( Fig. 10f–h ). Together, these data support the identification of ADAM10 as the specific metalloprotease targeting ephrinB2 in the absence of flotillin-1. In this paper we show that ephrinB2 ectodomain shedding and ephrinB2 levels are regulated by ADAM10, which is inhibited in the presence of endogenous flotillin-1. Furthermore, we present evidence that maintenance of ephrinB2 protein levels allows normal neural tube morphogenesis during Xenopus embryogenesis. Mice lacking ephrinB2 die in utero before embryonic day 11.5 owing to defects in the remodelling of the embryonic vascular system [30] , and ephrinB2 knockout mice display angiogenic defects in both arteries and veins [31] . Although neural tube closure defects have only been reported for ephrinB1-deficient mice [32] , there are other defects relating to cell–cell adhesion and morphogenesis that are revealed in engineered ephrinB2 null mice. For example, disruption of bi-directional signalling between ephrinB2 and EphB receptors impairs morphogenetic cell–cell septation and closure events during development of the embryonic midline. Mice lacking both EphB2/EphB3 forward signalling and ephrinB2 reverse signalling do not properly undergo midline fusion of the palate [33] . Moreover, ephrinB2 reverse signalling is critical to mediate ventral abdominal wall closure [33] . In the present study, we found that ephrinB2 plays a role in amphibian neural tube closure, and that it exerts its influence on the process of apical constriction, which is a cell shape change in the neural plate that bends the tissue, allowing for a tube to form [34] . In this paper, we have shown that specific loss of ephrinB2 affects apical constriction and the associated actin polymerization in Xenopus embryos ( Fig. 8c,d ), and that the loss of flotillin-1 phenocopies this effect ( Figs 7a,b and 8c,d ). Flotillin-1 is a scaffold protein associated with lipid rafts and we showed that it interacts with ephrinB2 and that they co-localize at the membrane, but how flotillin-1 might regulate ephrinB2 protein or signalling was not intrinsically obvious. The surprising finding that, in vivo , MO-mediated loss of flotillin-1 resulted in a dramatic decrease in ephrinB2, but not ephrinB1 or ephrinB3 ( Fig. 2d,g,h ), indicated a regulatory connection between these two proteins. The data showing that forced overexpression of ephrinB2 can rescue the neural tube closure defect induced by the loss of flotillin-1 confirmed that flotillin-1 was mediating its effect by regulating ephrinB2 levels ( Fig. 9a–c ). Moreover, using specific MOs that target ADAM10, or an ADAM10-specific inhibitor, clearly indicated that ADAM10 is the metalloprotease responsible for the substantial cleavage and loss of ephrinB2 in the absence of flotillin-1 ( Figs 4b,c; 5a,e and 6a–c ,). Further evidence was provided by functional assessments in vivo , where an ADAM10 MO rescued the neural tube closure defect induced by F1aMO ( Fig. 10a,b ). These data were also supported by experiments showing neural tube defects in embryos exogenously expressing ADAM10 ( Fig. 10c–e ). The planar cell polarity (PCP) signalling pathway has been shown to be a key signalling system for neural tube closure [34] , [35] , and ephrinBs have also been linked to the PCP pathway [36] , [37] . For example, it has been shown that ephrinB1 can activate PCP signalling and therefore promote the morphogenetic movement of retinal progenitors into the eye field [37] , and that ephrinB1 inhibits canonical Wnt signalling, unless cleaved by ADAM13 (ref. 11 ). EphrinB2 shares high homology with ephrinB1, particularly in the carboxy terminus that associates with the Wnt/PCP scaffold protein dishevelled, and is necessary for ephrinB1-mediated regulation of PCP signalling [36] , [37] . Thus, it may be possible that ephrinB2 mediates proper neural tube formation via the PCP pathway, and therefore that loss of flotillin-1 de-represses ADAM10 activity towards ephrinB2 in the neural tube, leading to inhibition of PCP signalling and impaired neural tube formation. Currently, how flotillin-1 inhibits ADAM10 activity towards ephrinB2 is still unclear. As we show here, flotillin-1 interacts with ephrinB2 ( Fig. 1a,b ), suggesting that the binding of flotillin-1 to ephrinB2 may inhibit ADAM10-mediated cleavage of ephrinB2. However, an ephrinB2 Δ60 mutant that displays a greatly reduced affinity for flotillin-1 when compared with wild type is also decreased in the absence of flotillin-1. Moreover, flotillin-1 does not associate with ADAM10 in our co-IP assays, indicating that flotillin-1 may indirectly inhibit ADAM10 activity through as yet unknown proteins. ADAM10 activity is regulated by several other proteins: for example, the immature form of ADAM10 is processed by other proteases such as furin, a calcium-dependent serine protease [38] and proprotein convertase 7 (ref. 39 ) to yield a mature active ADAM10. It has also been shown that several tetraspanins can regulate ADAM10 trafficking from the endoplasmic reticulum to the cell surface and promote maturation [40] , while tissue inhibitor of metalloproteinases inhibit ADAMs [41] . Therefore, it is possible that flotillin-1 may indirectly regulate ADAM10 through one of these regulators. Another possibility is that an association with flotillin-1 may sterically hinder or physically block an interaction between ephrinB2 and ADAM10. This may be less likely since ADAM10 targets the ephrinB2 ectodomain for cleavage, while flotillin-1 interacts with the intracellular domain of ephrinB2. Alternatively, it is also possible that flotillin-1 may regulate ephrinB2 localization in specific microdomains that are spatially separate from ADAM10 microdomains in the plasma membrane. Data consistent with these possibilities are observed in MG132-treated embryos that co-express a protease-deficient mutant of ADAM10 and wild-type ephrinB2 in the presence of F1MO. IPs from these embryos show a marked increase in the amount of ADAM10 that associates with ephrinB2 when compared with controls ( Fig. 5f ). The data in Fig. 1e (and the Supplementary Movie 1 ) support the concept that flotillin-1 and ephrinB2 can co-localize at the plasma membrane, but these data are not sufficient to indicate that these proteins are found in or transit between microdomains. Such evidence will require the development of appropriate antibodies to examine endogenous proteins under high-resolution microscopy. The role of Eph receptor engagement of the ephrinB2 ligand in the initiation and regulation of this process remains to be elucidated. We generated an ephrinB2 C100Y mutant that is compromised in EphB4 receptor binding [42] , [43] ( Supplementary Fig. 5a ), and found that this mutant also displays markedly reduced protein levels in the presence of the F1aMO ( Supplementary Fig 5b ). In addition, use of MOs against several possible cognate Eph receptors (gifts from Francois Fagotto) including EphA4, EphB1, EphB2 and EphB4 did not affect the reduction in exogenously expressed wild-type ephrinB2 caused by the F1aMO ( Supplementary Fig. 5c ). Moreover, while the EphB receptor MOs did not have an effect on the reduction in exogenously expressed wild-type ephrinB2 protein levels caused by overexpression of ADAM10, the EphA4 MO prevented a reduction in ephrinB2 levels ( Supplementary Fig. 5d ). However, there are limits to this analysis since the efficiency of the Eph MOs is not clear because of lack of appropriate antibodies for the Xenopus system. It has been reported that flotillin-1 regulates caveolin-1, since short interfering RNA-mediated downregulation of flotillin-1 expression disrupted lipid raft-mediated endocytosis and also substantially decreased caveolin-1 levels in human intestinal epithelial cells [44] . Similar to ephrinB2, the decrease in caveolin-1 expression appeared to be specific for flotillin-1 knockdown and suggested that flotillin-1 regulates caveolin-1 levels by preventing its degradation. Although flotillins and caveolins do not physically interact, and occupy distinct microdomains of the plasma membrane [45] , [46] , they may cross-talk or cooperate in regulating different segments of the endocytic process [47] , [48] . Another possibility is that flotillin-1 not only regulates both ephrinB2 cleavage and stability but also regulates N-cadherin. Recently, it has been reported in epithelial cells that flotillin microdomains are required for N-cadherin stabilization at cell–cell junctions [49] , and ADAM10 has been shown to be responsible for the constitutive and regulated shedding of N-cadherin expression at the cell surface in neuronal cells and fibroblasts [50] . Thus, it is possible that N-cadherin, similar to ephrinB2, is regulated by flotillin-1 via ADAM10-mediated cleavage, and also contributes to the neural tube phenotype. Further studies will be needed to elucidate precisely how flotillin-1 inhibits ADAM10 activity towards ephrinB2. Plasmids and reagents A full-length Xenopus laevis ephrinB2 complementary DNA clone was obtained from Thermo Scientific (GenBank ID: BC057724). HA- or Flag-tagged ephrinB2, B2 11MT -HA, ephrinB2 Δ60 -HA and ephrinB2 TM-Cyto- HA were generated by PCR and subcloned into either pCS2+ or pCS107. B1B2-HA and B2B1-HA were constructed by subcloning of ephrinB1 or ephrinB2 ectodomains that were generated by PCR into ephrinB1 TM-Cyto or ephrinB2 TM-Cyto clones. EphrinB2 Δjuxta , ephrinB2 Δ168–177 , ephrinB2 Δ182–194 , ephrinB2 Δ197–218 and ephrinB2 C100Y clones were generated by QuickChange Site-Directed mutagenesis (Agilent). Xenopus laevis flotillin-1a and flotillin-1b cDNA clones [17] were gifts from SA Moody, and HA- or Flag-tagged flotillin-1a, flotillin-1b, flotillin-1a ΔUTR and flotillin-1b ΔUTR were generated by PCR and subcloned into either pCS2+ or pCS107. X. laevis HA-tagged ADAM10 and ADAM17 cDNA clones were gifts from S Wei, and DW DeSimone and V5-tagged ADAM10 and ADAM17 were generated by PCR and subcloned into pCS107 and pCS2+. ADAM10PD-V5 was generated by site-directed mutagenesis to convert the consensus active site (HEXGHXXGXXHD) to (HEXGDXXAXXYA). pCS-tmEphB4 clones [51] were kindly shared by A W Brändli, and nucleotides 1–1,791 were HA tagged and subcloned into pCS107 by PCR. B2MO, F1aMO, F1bMO, ADAM10 MO and ADAM17 MO were designed and synthesized with reverse complementary bases of designated sequences shown in Supplementary Fig. 6a,c,d,f,h (Gene Tools). ADAM13 MO is as described previously [52] . The broad-spectrum metalloprotease inhibitor, GM6001, was purchased from Calbiochem (catalogue number 364206), and BB-94 was obtained from TOCRIS Bioscience (catalogue number 2961). The ADAM10-specific inhibitor, GI254023X, was kindly shared by A Ludwig [53] . Embryo injections Xenopus embryos were obtained by standard methods [54] . Capped messenger RNA was synthesized using SP6 mMessage mMachine kit (Ambion) [55] , and injected into embryos in a volume of 1–10 nl using a pico-injector (Harvard Instruments). Forty nanograms of B2MO, 20 ng of F1aMO, 10 ng of F1bMO, 20 ng of ADAM10 MO, 10 ng of ADAM13 MO, 10 ng of ADAM17 MO, 10 ng of EphA4, EphB1, EphB2 or EphB4 MOs per embryo was injected at the two-cell-stage. For rescuing the MO effects, 0.15 ng of ephrinB2 11MT or 0.5 ng of flotillin-1 ΔUTR RNA was injected with each MO, unless otherwise indicated. For immunostaining, 0.15–0.3 ng of GFP RNA, 0.3 ng of ephrinB2 or 0.5 ng of flotillin-1 RNA was injected. Quantification of neural tube closure defects in ephrinB2 or flotillin-1 morphants in Figs 7 and 9a–c were as follows: embryos showing one centerline for the neural fold were counted as having closed neural tubes. If two lines of neural folds were visible, the embryo was regarded as embryos having a neural tube closure defect. At least three independent experiments were performed and error bars indicate s.d. Gap width between the neural folds of embryos was measured using ImageJ software on the dorsal side of the embryos. Apical constriction determination in embryos Analyses of apical constriction defects were performed [56] . In brief, to visualize cell shape, embryos were stained with anti-tubulin (green) antibody to outline the cell shapes and with anti-GFP (red) antibody to label the injected side at the neurula stage. Then the lengths of the apical surface and perimeter were measured based on anti-tubulin staining using ImageJ software. The average ratios of the apical surfaces to the perimeters among five different neuroepithelial cells on each side of the midline were calculated for five different embryos and the ratios were compared between the uninjected side and the MO-injected side. Immunoprecipitation and western blot analysis Immunoprecipitation and western blot analysis were performed as described previously with a minor modification [55] . In brief, lysates of HT-29 cells, oocytes or embryos were prepared with cold lysis buffer. Immunoprecipitations were conducted on HT-29 cell lysates or 15 oocyte/embryo equivalents at 4 °C for 4–16 h with the anti-HA, anti-Flag (Applied Biological Materials), anti-ephrinB2 (R&D systems AF496) or anti-His antibodies, and protein-A/G agarose (Santa Cruz Biotechnology). Immunoprecipitates were washed with either RIPA or lysis buffer three times. Immunoblotting was conducted using anti-Flag-horseradish peroxidase (HRP; Sigma), anti-HA-HRP (Roche), anti-ephrinB2 (Abcam 75868), anti-flotillin-1 (Santa Cruz Biotechnology SC74566), anti-ADAM10 (Abcam, ab1997) anti-Erk2 (Santa Cruz Biotechnology) or anti-V5 (Invitrogen) antibodies in 5% milk. Anti-Flag-HRP and anti-HA-HRP were diluted 1:2,000, anti-ephrinB2 and anti-flotillin-1 were diluted 1:1,000, anti-Erk2 was diluted 1:10,000, and anti-V5 was diluted 1:5,000. Full scans of western blots are presented in Supplementary Fig. 7 . Immunofluorescence microscopy Xenopus embryos were collected at stage 15–17 for apical constriction analysis and F-actin staining, and stage 9–10 for exogenous ephrinB2 staining. Embryos were fixed with Dents fixative (80% methanol, 20% dimethylsulphoxide) for 1 h at room temperature (RT). For F-actin staining, formaldehyde-glutaraldehyde (FG) fixative (3.7% formaldehyde, 0.25% glutaraldehyde, 0.1% Tween-20 in PBS) was used instead of Dents. If needed, embryos were embedded in 15% fish gelatin, frozen and sectioned using a cryostat, as described previously [57] . After incubation in blocking buffer (1% BSA, 20% goat serum in PBS) for 30 min at RT, samples were incubated with appropriate primary antibodies overnight at 4 °C. Then, embryos were washed three times with PBS for 5–10 min, and treated with the appropriate secondary antibody for 4 h at RT. Before imaging, embryos were washed three times with PBS. The following primary antibodies were used: mouse anti-α tubulin (Sigma, 1:400), rabbit anti-GFP (Abcam, 1:400), mouse anti-GFP (Roche, 1:400), mouse anti-HA (Applied Biological Materials, 1:400), mouse anti-flotillin-1 (BD Biosciences, 1:200) or mouse anti-Flag (Applied Biological Materials, 1:400). To visualize, Cy3-conjugated anti-rabbit IgG (Jackson Immuno Research Laboratories, 1:400), Alexa Fluor 488 anti-mouse IgG (Invitrogen, 1:400), or Alexa Fluor 594 anti-mouse IgG was added to the samples after washing. For F-actin staining, 4 U ml −1 of Texas Red-X phalloidin was added with the secondary antibody. Analysis of the total actin signal in neuroectoderm The integrated density of the neuroectoderm, which is indicated in third column of Fig. 8c , was determined using ImageJ software. The total actin intensity of the neuroectoderm is calculated by the equation: Total intensity of neuroectoderm=integrated density−(area × mean intensity of the background).The average mean intensity of the background is calculated from at least three different regions of the neurectoderm, and is set in the cell centre. Determination of ephrinB2 half-life Western blot analysis of stage 14–18 embryos previously injected with HA-tagged ephrinB2 RNA that was titrated to yield roughly equivalent ephrinB2 protein levels in the presence of the indicated MOs. The embryos were injected (10 nl of 75 μg μl −1 , into the archenteron cavity) and treated (7.5 μg μl −1 ) with CHX and only injected with GI254023X (10 nl of 1 mM) and incubated for designated hours. Western blot with anti-Erk2 antibodies was also performed for loading controls. The quantification of the data from three independent experiments is displayed; error bars show positive value of s.d. Determination of cell surface ephrinB2 MOs were injected in both cells of two-cell-stage embryos and the ADAM10 inhibitor GI254023X (10 nl of 1 mM) and proteosomal degradation inhibitor MG132 were injected into the blastocoel at stage 9 and archenteron at stage 14, respectively. The dorsal axial region (neural fold) was excised at stage 16–18 and treated with sulfo-NHS-LC-biotin (1 mg ml −1 , Pierce # 21335) in 1XMMR at 4 °C for 30 min to label cell surface proteins. Then the excess biotin was washed with 10 mM glycine in 1X Marc's Modified Ringer's (MMR) three times and the explants were immediately harvested and lysed. Total cell surface proteins were precipitated with streptavidin sepharose and ephrinB2 was detected with ephrinB antibody (Santa Cruz Biotechnology, C-18). To determine the total level of ephrinB2, western analysis was performed on direct lysates, and Erk2 was immunoblotted as a loading control. Co-localization in embryos RNAs of Flot1a-EGFP and ephrinB2-mCherry were radially injected into two-cell-stage embryos at the equatorial region. Injected embryos were bisected at stage 8 along the median plane and transferred to a glass-bottom culture dish filled with Danilchik medium, with the sectioned surface contacting a fibronectin-coated coverslip. Another coverslip was overlayed on the specimen and supported by grease at four corners. The GFP and mCherry signals were detected by time-lapse confocal microscopy using a Zeiss LSM510 with double channel and a single track. How to cite this article: Ji, Y. J. et al. EphrinB2 affects apical constriction in Xenopus embryos and is regulated by ADAM10 and flotillin-1. Nat. Commun. 5:3516 doi: 10.1038/ncomms4516 (2014).